Sequential growth of long DNA strands with user-defined patterns for nanostructures and scaffolds DNA strands of well-defined sequence are valuable in synthetic biology and nanostructure assembly. Drawing inspiration from solid-phase synthesis, here we describe a DNA assembly method that uses time, or order of addition, as a parameter to define structural complexity. DNA building blocks are sequentially added with in-situ ligation, then enzymatic enrichment and isolation. This yields a monodisperse, single-stranded long product (for example, 1,000 bases) with user-defined length and sequence pattern. The building blocks can be repeated with different order of addition, giving different DNA patterns. We organize DNA nanostructures and quantum dots using these backbones. Generally, only a small portion of a DNA structure needs to be addressable, while the rest is purely structural. Scaffolds with specifically placed unique sites in a repeating motif greatly minimize the number of components used, while maintaining addressability. This combination of symmetry and site-specific asymmetry within a DNA strand is easily accomplished with our method. Long strands of DNA with controlled sequence are extremely valuable, information-rich molecules. From customized genes [1] to high-density data storage tools [2] to backbones for structurally diverse nanostructures [3] , [4] , [5] , [6] , there is a tremendous interest in developing synthetic protocols for the production of sequence-defined DNA that is longer than what conventional solid phase synthesis can achieve (>200 bp). For many applications, the entire product must be completely sequence-unique to maximize information density. However, in some cases, repeating patterns of sequence are desirable. Structural proteins like elastin, collagen and silk often contain repeating peptide motifs, and are therefore translated from repeating DNA sequences [7] . This has sparked an interest in engineered ‘protein-polymers,’ developed with similar motifs from repeating DNA to optimize structural properties [8] , [9] . DNA is also a versatile self-assembly material, with promise in fields ranging from nanoelectronics to drug delivery [10] , [11] . Often, a long DNA strand serves as a continuous backbone, tying together many shorter components into a robust nanostructure (DNA origami), with size and addressability dictated by this backbone [3] . This backbone is typically derived from a bacteriophage and is completely unique in sequence along its length. However, this imposes a significant cost limitation, as each design requires hundreds of different staple strands for assembly. In many cases, most of the DNA scaffold is used merely for structural definition, while only a small portion is the ‘working area’, and needs to be of unique sequence to position cargo. In principle, if these purely ‘structural’ areas were made of repeating sequences, this would greatly minimize the number of component strands and the cost of the assembly. However, in practice, this would require the construction of ‘designer’ DNA strands that contain precisely placed unique sites within repeating DNA motifs, which is difficult to achieve with conventional techniques. Current methods to produce long, patterned DNA fall into three main categories: stepwise or parallel ligations, usually with intervening purification [12] , [13] , [14] or enzymatic selection [15] , overlap extension or related polymerase chain reaction (PCR) techniques, using many short overlapping fragments [1] , [16] , [17] , and enzymatic amplifications like rolling circle amplification (RCA) [7] , [18] . The first provides full control over the final product, but is time consuming and labour intensive. Overlap extension PCR is much faster and finds extensive use in gene synthesis, but is not compatible with sequence symmetry as the overlapping fragments would become scrambled. In contrast, RCA is only compatible with full sequence symmetry. This prevents the introduction of uniquely addressable sites within the pattern. As well, it yields a wide distribution of product lengths. We were therefore interested in developing a facile new strategy to generate long, single-stranded DNA rapidly and with full control over the sequence pattern and monodispersity. Here we describe a temporally controlled strategy to build patterned DNA backbones. With a small set of building blocks, we use order of addition and in situ ligation to grow products with various patterns of sequence domains. The full-length target product is then enriched using PCR, and converted to an addressable, single-stranded backbone using an isolation step with magnetic beads. The entire process can be done in a single day, using basic molecular biology instrumentation. Using this strategy, we generated monodisperse products with a range of sizes (480–1,058 bases) and sequence patterns, and demonstrated their ability to serve as addressable backbones for building DNA nanostructures or organizing cargo. With temporal control, a large set of diverse products could be produced rapidly from the same library of building blocks. Complexity in DNA nanotechnology is usually obtained by using unique strands and sequences to define different parts of a structure. In contrast, the oligonucleotides themselves are synthesized using time and order of addition, to grow complex sequences from four simple building blocks (automated solid-phase phosphoramidite synthesis). This mechanism allows a user to generate any arbitrary oligonucleotide sequence rapidly and from the same simple starting materials, and is responsible for the widespread use of synthetic DNA throughout the biological sciences. This manuscript applies the same concept of temporal control to create sequence patterns, but using entire DNA duplexes as the building blocks rather than single bases. As such, much larger products become accessible, which can be used to generate higher order assemblies and introduce new complexity into DNA nanotechnology without increased cost. This technique could open the door to easily accessible ‘designer’ DNA templates for the rapid generation of complex libraries of DNA nanostructures in a practical, cost-efficient manner. Sequential growth of long DNA strands To create temporally controlled patterns with DNA, we designed a small number of complementary duplex building blocks ( Fig. 1a ). Each one contains a sequence domain that can be included within the overall pattern (e.g., block A introduces sequence domain A ). Thus, on the basis of the order of addition, we hoped to generate various patterns of these sequence domains. Each building block is composed of a sense strand (for example, A1, dark red), with the desired sequence domain, and a carrier strand (for example, A2, light red), used to introduce addressability by placing sticky end overhangs at either end of the duplex. Building blocks A and B, as well as terminal versions that could only extend in one direction (A P and B P ), were synthesized. They contain sequence domains A and B respectively, with 42 bases each, and sticky ends that have 10 bases. Initially, we began by targeting a simple A-B alternating pattern. Beginning from A P , sequential addition of B, then A, then B and finally A again should produce a pentameric system, with an alternating A-B-A-B-A sequence domain pattern in the sense direction ( Fig. 1b ). The product would be nicked, but was expected to be stable under ambient conditions due to DNA base pairing of the sticky ends (expected melting temperature ∼ 40 °C under our conditions). As shown in Fig. 1b , however, sequential growth in this manner did not yield the expected pentameric product. Instead, a smear was observed by native agarose gel electrophoresis (AGE, lane 5). This is consistent with the building blocks rearranging during stepwise growth, scrambling the intended pattern. 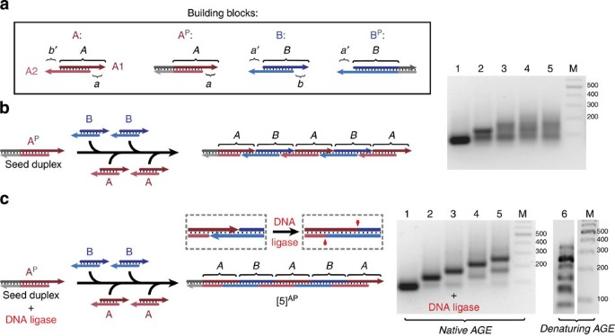Figure 1: Temporal control of DNA growth. (a) Each building block is composed of a sense strand (top, darker colour, for example, A1) with the desired sequence domain (A) and a carrier strand (bottom, lighter colour, for example, A2). The building block has sticky end overhangs at either end (for example, sequencesaandb’) for hybridizing to other building blocks. Four basic building blocks were used: A and B (internal, sequence domainsAandB, respectively) and APand BP(terminal, sequence domainsAandB, respectively). (b) Temporal growth of a pentamer via hybridization only, characterized by native agarose gel electrophoresis (AGE). Lane 1: AP, lane 2: AP+B, lane 3: AP+B+C, lane 4: AP+B+A+B, lane 5: AP+B+A+B+A. (c) Temporal growth of [5]APusingin situligation, characterized by native AGE (lanes 1–5, same lane assignments). Denaturing [5]AP(lane 6) reveals the presence of both the full-length covalent product and shorter truncated products as a result of incomplete ligation. Figure 1: Temporal control of DNA growth. ( a ) Each building block is composed of a sense strand (top, darker colour, for example, A1) with the desired sequence domain ( A ) and a carrier strand (bottom, lighter colour, for example, A2). The building block has sticky end overhangs at either end (for example, sequences a and b’ ) for hybridizing to other building blocks. Four basic building blocks were used: A and B (internal, sequence domains A and B , respectively) and A P and B P (terminal, sequence domains A and B , respectively). ( b ) Temporal growth of a pentamer via hybridization only, characterized by native agarose gel electrophoresis (AGE). Lane 1: A P , lane 2: A P +B, lane 3: A P +B+C, lane 4: A P +B+A+B, lane 5: A P +B+A+B+A. ( c ) Temporal growth of [5] AP using in situ ligation, characterized by native AGE (lanes 1–5, same lane assignments). Denaturing [5] AP (lane 6) reveals the presence of both the full-length covalent product and shorter truncated products as a result of incomplete ligation. Full size image However, when this sequential growth was performed in the presence of DNA ligase, scrambling was suppressed by covalently trapping each new building block as it was introduced. As shown in Fig. 1c , the same pentameric A-B-A-B-A pattern ([5] AP , 248 bp) was easily generated in fairly high yield ( ∼ 45% based on weighted band intensity) with this in situ ligation strategy. Note that we use the nomenclature [N] to represent products with N alternating sequence domains. The ‘AP’ superscript denotes that the product was grown from the A P seed duplex. A number of parameters were optimized to achieve the results in Fig. 1 , including the phosphorylation of individual component strands, ligase concentration, incubation times and stoichiometry (see Supplementary Fig. 1 ). Both reactions ( Fig. 1b,c ) used identical, optimized conditions save for the addition or omission of DNA ligase, emphasizing the importance of in situ ligation for promoting efficient temporal growth. This effect was observed despite the fact that ligation does not proceed with 100% efficiency. As shown in Fig. 1c (lane 6), denaturing [5] AP to observe the component strand sizes reveals a distribution of products from the intended pentamer all the way down to monomers. This is likely due to a combination of failed phosphorylation and ligation steps during growth, as neither process is expected to proceed quantitatively. On the basis of lanes 1–5, however, ligation is frequent enough to trap the majority of incoming building blocks as intended. From the denaturing analysis in Figs 1c and 2d (below), we have estimated the ligation efficiency at ∼ 85% per nicked site. Incoming building blocks introduce two new sites, but ligating just one of them is likely sufficient to anchor them in place. At 85% efficiency, > 97% of building blocks would ligate at least once and become trapped in place. This explains the apparent contrast between lanes 5 and 6 in Fig. 1c , and shows that [5] AP is composed of both fully covalent and partially nicked products. As discussed below, however, we have developed a strategy to enrich and isolate the full-length target strands from this mixture. Using this strategy, even very low yields of fully ligated product are sufficient to generate usable material. 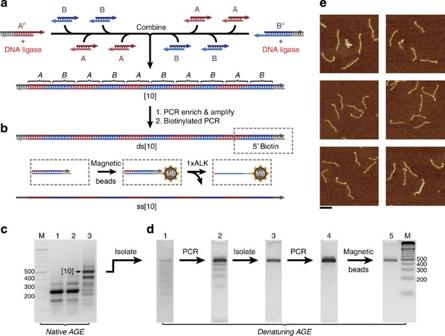Figure 2: Temporal growth and enrichment of an alternating decameric product. (a) Schematic procedure for temporal growth of [10]. (b) Schematic procedure for isolating ss[10] using magnetic beads. A biotinylated reverse primer yields a 5′ biotin on the antisense strand. Incubation with streptavidin-coated magnetic beads followed by alkaline denaturation allows the isolation of ss[10] from the PCR product mixture. (c) Growth characterized by native AGE. Lane 1: [5]AP, lane 2: [5]BP, lane 3: [5]AP+[5]BP(= [10]).c, Denaturing AGE characterization of [10] and subsequent enrichment of the non-nicked product ds[10], and isolation of the single-stranded product ss[10]. Lane 1: [10], lane 2: [10] amplified by PCR, lane 3: isolated ds[10], lane 4: ds[10] amplified by PCR, lane 5: ss[10] isolated using magnetic beads. (d) AFM characterization of ds[10], scale bar is 100 nm. Figure 2: Temporal growth and enrichment of an alternating decameric product. ( a ) Schematic procedure for temporal growth of [10]. ( b ) Schematic procedure for isolating ss[10] using magnetic beads. A biotinylated reverse primer yields a 5′ biotin on the antisense strand. Incubation with streptavidin-coated magnetic beads followed by alkaline denaturation allows the isolation of ss[10] from the PCR product mixture. ( c ) Growth characterized by native AGE. Lane 1: [5] AP , lane 2: [5] BP , lane 3: [5] AP +[5] BP (= [10]). c , Denaturing AGE characterization of [10] and subsequent enrichment of the non-nicked product ds[10], and isolation of the single-stranded product ss[10]. Lane 1: [10], lane 2: [10] amplified by PCR, lane 3: isolated ds[10], lane 4: ds[10] amplified by PCR, lane 5: ss[10] isolated using magnetic beads. ( d ) AFM characterization of ds[10], scale bar is 100 nm. Full size image With an optimized strategy in hand, we next targeted a larger product. By growing [5] AP and [5] BP in parallel and then combining them, the decameric product [10] could be produced rapidly (30 min, room temperature) and in reasonable yield ( ∼ 30% based on weighted band intensity, Fig. 2c ). This product is 480 bp in length, has five A and five B alternating sequence domains and is blunt at both ends. Product amplification Product [10] was grown in bulk and isolated by 2% native AGE. As expected, denaturing analysis of [10] revealed that it was highly nicked, such that only a small fraction of the strands comprising it were the full-length, intended product ( Fig. 2d , lane 1). A simple strategy to overcome this and enrich the target strand was developed. A P and B P contain unique end-capping sequences, shown in grey above. Only fully ligated products will contain both of these sequences on the same strand, while any nicked byproducts would contain only one or neither. Thus, amplifying [10] by PCR with primers that match these end sequences would enrich full-length products exponentially, while nicked ones would amplify only linearly or not at all. A complication of this strategy is that nicked products could act as non-specific primers for each other, since Taq polymerase will act on any recessed 3′ DNA. Indeed, this phenomenon, termed the ‘concatemer chain reaction’ , has been used to generate long, concatemeric ladders of DNA products from a set of partially complementary strands [19] . To minimize interference by concatemer chain reaction, relatively stringent annealing conditions were used during PCR cycling to suppress any lower affinity, unintended priming events (see Supplementary Discussion ). As shown in Fig. 2d , this was successful in favouring the full-length product for enrichment and subsequent isolation. This strategy was used to enrich [10], followed by isolation from denaturing AGE. Subsequent analysis confirmed that this new product, ds[10], was composed entirely of full-length strands ( Fig. 2d , lane 3). Once isolated, ds[10] could be reamplified by PCR if needed to generate large quantities of the double-stranded product for subsequent experiments ( Fig. 2d , lane 4). The full-length product was isolated with a significant amplification (1–1.5 μg of ds[10] from 16 ng of nicked [10], or a nominal ‘yield’ of >500% when comparing moles of ds[10] recovered per mole of A P used during the initial growth reaction). This procedure more than makes up for losses due to low ligation efficiency: the target strand can be recovered even if it is a very small fraction of the original growth reaction. Atomic force microscopy (AFM) of ds[10] ( Fig. 2e ) revealed an average length of 163.6±7.0 nm (from 41 features), matching the expected value of 163.2 nm for B-form DNA. Conversion to a single-stranded DNA backbone To make use of temporally grown sequence patterns, we needed a method to convert double-stranded products to their single-stranded analogues, which can serve as templates for organizing other structures through complementary base pairing. Our products were made with two different strategies in mind for converting them to single-stranded versions: strand displacement amplification [20] (see Supplementary Discussion ) or PCR followed by separation with magnetic beads. PCR gave better yields and was therefore used in all subsequent experiments. We carried out PCR amplification using a biotinylated reverse primer, thus allowing the subsequent removal of the antisense strand using streptavidin-coated magnetic beads ( Fig. 2b ). Biotinylated PCR products were bound to magnetic beads, washed and then denatured with alkaline buffer. This released the single-stranded product ss[10] into the supernatant, from which it could be recovered by ethanol precipitation ( Fig. 2d , lane 5). Owing to the amplification step, 1–2 μg of ss[10] could be recovered from just 4 ng of ds[10]. To demonstrate the generality of our approach, we also made a library of other products with different numbers, patterns and lengths of building block domains, all in similar yields (see Supplementary Table 2 ). As the yield is maintained with increasing length of the product strand (for example, 1,058 bases), we anticipate being able to form products approaching the length of typical bacteriophage scaffolds used in DNA origami. Site-specific modification of sequence To confirm that our temporal strategy actually controlled the sequence pattern of the resulting product, we next site-specifically incorporated a recognition site (5′-TCTAGA-3′) for the restriction enzyme XbaI, at two different positions in two decameric products. Building block X (composed of X1 and X2) was used in place of B at either the second or sixth position beginning from A P ( Fig. 3a ). On isolation, PCR enrichment and purification, this yielded the products ds[10] XbaI-2 and ds[10] XbaI-6 ( Fig. 3b ). As shown in Fig. 3c , digestion of each product with XbaI restriction enzyme gave the expected fragment sizes based on the location of the restriction site. This confirms that the temporal strategy employed here, followed by PCR enrichment and purification, allows external control over the sequence domain pattern of the resulting product. 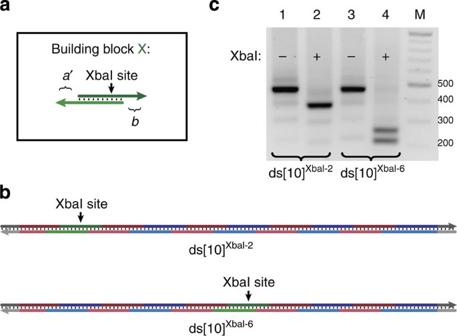Figure 3: Restriction assay to confirm temporal control over sequence domain pattern. (a) Building block X could be used in place of B and contained an XbaI recognition site. (b) Location of XbaI restriction sites in ds[10]XbaI-2and ds[10]XbaI-6based on temporal control. (c) Native AGE characterization of products ds[10]XbaI-2and ds[10]XbaI-6with and without XbaI digestion, showing the expected fragments in each case (93 and 387 bp for ds[10]XbaI-2, 219 and 261 bp for ds[10]XbaI-6). Note that the 93 bp fragment from ds[10]XbaI-2was not visible due to poor staining efficiency. Lanes as marked. Figure 3: Restriction assay to confirm temporal control over sequence domain pattern. ( a ) Building block X could be used in place of B and contained an XbaI recognition site. ( b ) Location of XbaI restriction sites in ds[10] XbaI-2 and ds[10] XbaI-6 based on temporal control. ( c ) Native AGE characterization of products ds[10] XbaI-2 and ds[10] XbaI-6 with and without XbaI digestion, showing the expected fragments in each case (93 and 387 bp for ds[10] XbaI-2 , 219 and 261 bp for ds[10] XbaI-6 ). Note that the 93 bp fragment from ds[10] XbaI-2 was not visible due to poor staining efficiency. Lanes as marked. Full size image Note that the faint upper and lower bands in Fig. 3c only show up under native conditions, and are therefore likely phase-shifted or looped duplexes. Owing to the repeating sequence of these products, the two component strands can rehybridize partially out of phase with each other after denaturing purification. When a single-stranded product is desired anyway this is not a problem, as the complementary strand will be removed. To further test the sequence fidelity of our strategy, we built a fully asymmetric 452 bp product for DNA sequencing (‘L[4]’, see Supplementary Information ). L[4] was inserted into the pUC119 plasmid using restriction digestion and ligation, and then transformed into DH5α E. coli to generate a clonal product. Sanger sequencing found an error rate of 0.5%, which includes contributions from solid-phase synthesis of the component strands ( ∼ 1% error rate [21] ) and the polymerase used through two 30-cycle amplifications ( ∼ 0.01% error rate per cycle, or ∼ 0.6% overall). Using a high-fidelity DNA polymerase and more robustly purified starting oligonucleotides could further increase this level of accuracy by several orders of magnitude. Note that L[4] was made asymmetric to simplify sequencing, as repeating sequences are difficult to analyse. Temporally grown strands as scaffolds for nanotubes One of the applications for these products is as addressable backbones in DNA nanostructures. Work by us [22] and other groups [5] , [23] has already shown that continuous template strands can help to augment the structural control and biological stability of the resulting products. The repeating A and B sequence domains of ss[10] were chosen to match the binding sites of DNA nanotube rungs that we have previously described (UA and UB) [6] . As such, they could be used as a backbone to produce DNA nanotubes whose length and longitudinal pattern are defined by the template strand ( Fig. 4a ). On incubating ss[10] with rung units UA and UB, a discrete low mobility band was observed by AGE ( Fig. 4b , lane 2), representing a nanotube with ten alternating rungs (NT[10]). The sharpness of this band is very different from the diffuse or non-penetrating bands that we previously obtained when nanotubes were templated on a backbone strand grown by RCA [24] , consistent with the monodispersity of ss[10]. 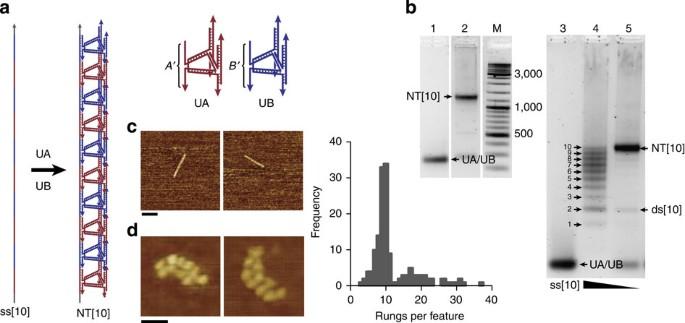Figure 4: Using single-stranded DNA to guide nanotube assembly. (a) Combining ss[10] with nanotube rungs UA and UB allows the production of monodisperse, patterned nanotubes NT[10]. (b) Assembly of NT[10] characterized by AGE. Lane 1: rungs UA+UB, lane 2: UA+UB+ss[10] (=NT[10]), lane 3: UA+UB, lane 4: UA+UB+5 eqv. ss[10], lane 5: UA+UB+1 eqv. ss[10]. Lane 4 shows nanotubes with 1–10 rungs bound, allowing proper band assignment for NT[10]. Lane 5 shows trace amounts of ds[10] present in ss[10]. (c) NT[10] characterized by AFM without rinsing, revealing extended nanotubes 146.2±18.6 nm in length, but limited structural detail. Scale bar, 100 nm. (d) NT[10] characterized by AFM with extensive rinsing, revealing individually resolved rungs but a collapsed morphology. Scale bar, 50 nm. The histogram shows the number of rungs observed per feature from a large set of data. Figure 4: Using single-stranded DNA to guide nanotube assembly. ( a ) Combining ss[10] with nanotube rungs UA and UB allows the production of monodisperse, patterned nanotubes NT[10]. ( b ) Assembly of NT[10] characterized by AGE. Lane 1: rungs UA+UB, lane 2: UA+UB+ss[10] (=NT[10]), lane 3: UA+UB, lane 4: UA+UB+5 eqv. ss[10], lane 5: UA+UB+1 eqv. ss[10]. Lane 4 shows nanotubes with 1–10 rungs bound, allowing proper band assignment for NT[10]. Lane 5 shows trace amounts of ds[10] present in ss[10]. ( c ) NT[10] characterized by AFM without rinsing, revealing extended nanotubes 146.2±18.6 nm in length, but limited structural detail. Scale bar, 100 nm. ( d ) NT[10] characterized by AFM with extensive rinsing, revealing individually resolved rungs but a collapsed morphology. Scale bar, 50 nm. The histogram shows the number of rungs observed per feature from a large set of data. Full size image By combining rungs with excess ss[10], a ladder of ‘partially filled’ nanotubes could be generated (nanotubes with 1, 2, 3 and so on rungs per scaffold, Fig. 4b , lane 4), allowing proper band assignment. This confirmed that the single band in lane 2 was indeed NT[10], with five equivalents of each rung bound. Note that the single-stranded backbone contains a small fraction of the corresponding double-stranded product ( Fig. 4b , lanes 2 and 5). This is likely due to partial streptavidin–biotin dissociation during the magnetic bead isolation procedure, releasing a small amount of the antisense strand. The amount of double-stranded product varied from batch to batch, but was generally minor (<5%). As seen in Supplementary Fig. 8 , a genuine sample of ds[10] matches the byproduct band and does not interact with the rung units. We also characterized NT[10] by AFM, using two different sample preparation methods for this analysis. The first revealed extended nanotubes with an average length of 146.2±18.6 nm, matching the theoretical value of 142.8 nm ( Fig. 4c ). Note that the terminal priming regions of ds[10] do not contribute rung-binding sites, such that NT[10] is shorter than ds[10] and is expected to show more length variation based on whether or not the single-stranded tails are visible for a given feature. The low structural detail of these images also makes it difficult to assess contributions from salt deposits or surface-induced disassembly, which would introduce significant measurement errors for these very small structures. For a more robust analysis, a second procedure was used with substantial rinsing to remove salt deposits that might obscure the finer structural details. This allowed us to consistently observe nanotubes with sufficient resolution to differentiate and count individual rungs, rather than just observing the overall length ( Fig. 4d ). However, this also introduced a ‘collapsing’ deposition artefact in which nanotubes appeared as clusters of rungs, instead of extended arrays. We hypothesize that this is due to strong interactions with the mica and Mg 2+ counterions in our nanotube assembly buffer during drying. Indeed, we have observed that [10] and ds[10] aggregate when deposited with increasing Mg 2+ (see Supplementary Discussion ). Despite this drying effect, we were still able to count the number of rungs associated with each nanotube structure. As shown in Fig. 4d , this value clusters around 10 for NT[10], or less frequently, multiples of 10 (resulting from multiple clustered nanotubes). Deviations from the expected number of rungs are likely due to rearrangements during sample deposition and drying, as the gel studies show that NT[10] consists of exactly 10 rungs in solution. Temporally grown strands for quantum dot organization Extended DNA nanostructures have shown promise as structural scaffolds that can organize patterned arrays of cargo, with potential in plasmonics [25] , catalysis [26] , [27] , artificial light harvesting [28] and nanoelectronics [29] , [30] . These applications require fine control over the placement and order of specific functional groups, which can be challenging at the nanometre scale. Temporally grown DNA backbones offer a unique, practical solution to these requirements. By using a small set of starting materials and simply changing the order of addition in each case, user-defined, monodisperse templates can be rapidly generated in high yield and used to arrange cargo into nanoscale patterns. To demonstrate this potential, we organized streptavidin-coated quantum dots (STV-QDs, CdSe/ZnS core, ∼ 15 nm diameter including the STV shell) into a number of linear patterns, as shown in Fig. 5 . For this, we used single-stranded backbones ss[10], ss[10] XbaI-2 and ss[10] XbaI-6 that were generated using our temporal growth method. A mixture of five strands complementary to A , B , X and the priming regions (cA, cB, cX, cFor, cRev) could be selectively bound by the single-stranded backbones, creating duplex products ( Fig. 5a ). If one of these strands was biotinylated, then its location within the duplex would become a binding site for the STV-QDs. Using our biotinylated reverse primer cRevBio, for example, we could bind a quantum dot to one end of the duplex ( Fig. 5b ). In contrast, with biotinylated cXBio, we could direct binding to either the second or sixth position along the backbone, using the appropriate template strand ( Fig. 5c,d ). 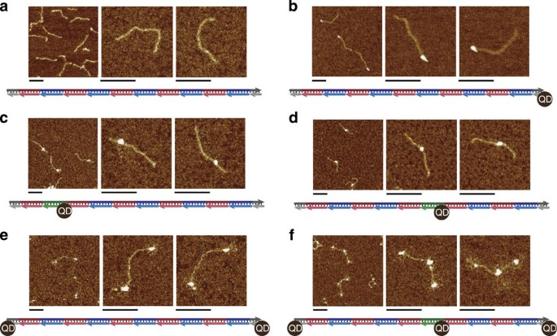Figure 5: Patterning quantum dot cargo with temporally grown backbones. (a) AFM characterization of backbone ss[10] with a mixture of complementary strands, creating a nicked duplex. (b) Backbone ss[10] with a mixture containing the 5′-biotinylated cRevBio and STV-QDs (= QDEnd). (c) Backbone ss[10]XbaI-2and a mixture containing cXBio (= QDInt). (d) Backbone ss[10]XbaI-6and a mixture containing cXBio (= QDMid). (e) Backbone ss[10] and a mixture containing cForBio and cRevBio (= QDDbl). (f) Backbone ss[10]XbaI-6and a mixture containing cForBio, cRevBio and cXBio (= QDTrpl). Scale bar, 100 nm. Figure 5: Patterning quantum dot cargo with temporally grown backbones. ( a ) AFM characterization of backbone ss[10] with a mixture of complementary strands, creating a nicked duplex. ( b ) Backbone ss[10] with a mixture containing the 5′-biotinylated cRevBio and STV-QDs (= QDEnd). ( c ) Backbone ss[10] XbaI-2 and a mixture containing cXBio (= QDInt). ( d ) Backbone ss[10] XbaI-6 and a mixture containing cXBio (= QDMid). ( e ) Backbone ss[10] and a mixture containing cForBio and cRevBio (= QDDbl). ( f ) Backbone ss[10] XbaI-6 and a mixture containing cForBio, cRevBio and cXBio (= QDTrpl). Scale bar, 100 nm. Full size image This trend can be expanded to multivalent patterns using several biotinylated strands, including site-specifically placed two ( Fig. 5e ) or three ( Fig. 5f ) quantum dots per backbone. This proof-of-concept system relies on the same attachment chemistry for each cargo (biotin-streptavidin), so multivalent patterns began to display cross-linking and higher order aggregation (see Supplementary Discussion ). Future systems could utilize orthogonal conjugation chemistries or attachment before assembly to overcome this limitation. The DNA structures presented here use a unique combination of sequence symmetry and site-specific asymmetry to organize their cargo into well-defined patterns at a minimal cost. Purely structural areas bind multiple copies of cA and cB to produce a rigid scaffold, while addressable areas are used to arrange cargo-binding strands within the resulting framework. Using temporal control we can quickly and easily programme different patterns of addressability, to arrange these binding sites precisely in space. DNA origami has become one of the gold standards for DNA nanostructures that are used as organizational scaffolds. It assembles consistently with low polydispersity and an addressable resolution of 6 nm [31] . However, this comes at the cost of hundreds of component strands, which can introduce a significant cost limitation. We are currently working to apply our temporal growth strategy, in combination with sequence symmetry, to develop simplified backbone strands for use in DNA origami assemblies. Most origami is used primarily for a small number of addressable sites, while the rest of the structure is merely filling space and providing robustness. We hypothesize that by replacing the traditional M13 bacteriophage backbone strand with a temporally grown, sequence symmetric product, we could generate origami structures from significantly fewer component strands (in multiple equivalents). Where addressability is required, the temporal strategy could be used to introduce unique sites selectively within the backbone. This would allow the rapid generation of an entire library of DNA origami scaffolds with molecular precision, from a very small set of building blocks. Current methods for producing long DNA can generate complete sequence symmetry or asymmetry, but user-defined combinations of the two are difficult to achieve. This work provides a simple, economic way to access such products for use in a wide range of nanotechnology applications. DNA nanotechnology has traditionally made use of large libraries of sequences and strands to generate complexity in a DNA structure. By relying on a unique sequence for each programmed interaction, one can define exactly where a component strand will end up within the final product. For many specific applications, however, this level of addressability is unnecessary. When using a nanostructure to organize two or three specific molecules into a well-defined pattern, for example, there is no need for the rest of the scaffold to be completely unique. This has provided motivation to introduce symmetry into such systems, such that a small number of repeating components can be used to provide the structural component. To retain addressability where needed, however, one must be able to selectively reintroduce asymmetric sites. This manuscript has described a method to generate DNA with arbitrary patterns of sequence using a temporal control. Simply by adjusting the order of addition, a small set of building blocks can be organized into diverse patterns, which can include both symmetric regions and unique sites, all under temporal control. This strategy is reminiscent of the solid-phase synthesis method used for making oligonucleotides, in which four basic building blocks (nucleoside phosphoramidites) are arranged into complex DNA sequences based on the cycle of additions. Our temporal growth approach relies on the use of an in situ ligation strategy to covalently trap each new building block as it is introduced. The desired product can then be isolated and enriched using PCR. One of the advantages of working with DNA is its biological nature; it is compatible with a wide range of enzymatic manipulations, allowing nature to do part of the work when using it. PCR not only enriched the desired product, but also allowed us to generate it in large quantities from fairly small-scale growth reactions, even if the original yield was poor. Once isolated, the single-stranded products generated by this strategy are capable of scaffolding other DNA nanostructures, or organizing cargo into user-defined patterns. This level of control, and the ability to combine symmetric and addressable regions within a DNA backbone, will allow the generation of highly complex DNA nanostructures from a small set of simple components, making DNA nanotechnology a more practical option for nanoscale patterning. Long strands of sequence-controlled DNA are used in other applications, as well, including customized gene synthesis and data storage. While these typically use completely asymmetric sequence, there could be specific cases where they might stand to gain from the basic methodology developed here, such as generating structural peptides with repeating motifs. Temporal growth Component strands were adjusted to 10 μM each and phosphorylated using OptiKinase (New England Biolabs) at 37 °C for 30 min, followed by 10 min at 75 °C to inactivate the enzyme. The double-stranded DNA building blocks were formed by combining complementary phosphorylated component strands (for example, A1 and A2), and adding an equal volume of 2xQL buffer (132 mM Tris-HCl, 20 mM MgCl 2 , 2 mM DTT, 2 mM ATP, 15% w/v PEG6000, with a pH of 7.6). These duplex stock solutions were then sequentially combined in the desired order (for example, A P , then B, then A and so on) in solution at room temperature, allowing 5 min of incubation time between each new addition. Once two building blocks were present, QuickLigase (New England Biolabs) was added to a concentration of 9.6 U μl −1 , followed by a 5 min incubation. Typical growth reactions used 75 pmol per addition, but could be scaled up or down. Longer products were grown in two halves (one from A P and one from B P ) and then combined, to maximize speed and yield. The desired product was isolated by native AGE using a QIAquick Gel Extraction Kit (Qiagen). PCR enrichment and isolation PCR was carried out in 40 μl batches, using the MyTaq Hot Start optimized PCR kit (CedarLane Laboratories), with 4 ng of template, 0.625 μM of each primer and 2 U of MyTaq HS Polymerase. An initial denaturation of 1 min at 95 °C was followed by 30 cycles of 95 °C for 15 s, 65 °C for 15 s, 72 °C for 10 s, for a total run time of ∼ 30 min. Typically four batches were run simultaneously, supplemented to 1 mM EDTA and then 1 × ALK (30 mM NaOH, 1 mM EDTA), and purified via 3% alkaline AGE. Products were analysed by 3% alkaline AGE and AFM (see Supplementary Discussion for details). Sequence control A variety of lengths and patterns were generated, with 4–14 sequence domains of different sizes (42 or 101 bases). Site-specific placement of building block X was confirmed using a restriction digestion assay. Products (200 ng) were exposed to 1 U of FastDigest XbaI (Thermo Scientific) for 2 h at 37 °C, and analysed by native AGE, revealing the expected fragment sizes for the target position of X. Generating single-stranded products PCR was carried out as above but with a biotinylated reverse primer. Products were treated with a QIAquick PCR Purification Kit (Qiagen), and then adjusted to a composition of 75 mM NaCl, 7.5 mM sodium citrate and pH 7.0. They were then incubated with 100 μl of Streptavidin MagneSphere paramagnetic particles (Promega) for 1 h with gentle inversion and exchanged to 1 × ALK buffer to denature the base pairing. After 15 min, the supernatant was recovered and ethanol precipitated, yielding single-stranded product. Nanotube assembly Nanotube rungs were prepared by combining their component strands to a final concentration of 436 nM in 1 × TAMg buffer (45 mM tris(hydroxymethyl)-aminomethane, 7.6 mM MgCl 2 , pH 8.0 with acetic acid), and annealing them from 95 °C to room temperature over 45 min. These were combined with 0.8 equivalents of single-stranded backbones and annealed from 44 °C to room temperature over 45 min, to maximize binding. This small excess of rungs was used to ensure full loading of nanotubes, regardless of potential stoichiometric or pipetting errors. Nanotubes were characterized by 2% native AGE and AFM (see Supplementary Discussion for details). Patterning quantum dots Single-stranded backbones were combined with a mixture of short strands complementary to their various sequence domains, using a slight excess (1.2x) to avoid stoichiometric errors. These products were assembled at 36 nM in 1 × TSC (9.75 mM Tris-Cl, 100 mM NaCl, pH 8.5), and annealed from 44 °C to room temperature over 45 min. Complementary mixtures with selected biotinylated strands were used, in combination with the choice of backbone sequence, to create different patterns of biotin binding sites. A twofold excess of Qdot 525 streptavidin-coated quantum dots (Invitrogen) was then added, and incubated at room temperature for >3 h. Products were analysed by native AGE and AFM (see Supplementary Discussion for details). How to cite this article: Hamblin, G. D. et al. Sequential growth of long DNA strands with user-defined patterns for nanostructures and scaffolds. Nat. Commun. 6:7065 doi: 10.1038/ncomms8065 (2015).